Mouse urinary peptides provide a molecular basis for genotype discrimination by nasal sensory neurons Selected groups of peptides, including those that are presented by major histocompatibility complex (MHC) proteins, have been proposed to transmit information to the olfactory system of vertebrates via their ability to stimulate chemosensory neurons. However, the lack of knowledge about such peptides in natural sources accessible for nasal recognition has been a major barrier for this hypothesis. Here we analyse urinary peptides from selected mouse strains with respect to genotype-related individual differences. We discover many abundant peptides with single amino-acid variations corresponding to genomic differences. The polymorphism of major urinary proteins is reflected by variations in prominent urinary peptides. We also demonstrate an MHC-dependent peptide (SIINFEKL) occurring at very low concentrations in mouse urine. Chemoreceptive neurons in the vomeronasal organ detect and discriminate single amino-acid variation peptides as well as SIINFEKL. Hence, urinary peptides represent a real-time sampling of the expressed genome available for chemosensory assessment by other individuals. While in humans the visual system discriminates individuals [1] , mice, as nocturnals, rely on olfactory cues released by bodily secretions in social behaviours such as mate choice, territorial scent marking and aggression [2] , [3] , [4] , [5] . Mice may identify conspecifics by both the main olfactory epithelium as well as the vomeronasal organ (VNO), responding to bodily secretions such as urine. Individual recognition requires a specific scent signature, which may entail qualitative or quantitative variation in volatile and/or involatile molecules. The earliest hypothesis trying to explain individual recognition in mice during mating postulated a connection between olfaction and the immune system represented by the polymorphic genes of the major histocompatibility complex (MHC, also called H2 in the mouse) [6] , [7] . MHC disassortative mating is considered as a mechanism to avoid inbreeding and to increase disease resistance in the progeny (for a review, see Slev et al . [8] ). Although this proposal stimulated extensive experimental and theoretical work, unravelling the underlying molecular mechanisms proved to be difficult. Two major mechanisms for explaining the functional link between the MHC as defined by the MHC class I molecules and relevant olfactory cues have been proposed in mice. In the first one, the MHC has been considered to influence the volatile composition of urine, as demonstrated by habituation, training and other tests with MHC congenic or mutant inbred strains [9] , [10] , [11] , [12] , [13] , [14] , [15] . Analysis of urinary volatiles of single inbred mice showed considerable variation in the abundance of certain volatiles. However, no qualitative and only negligible quantitative variations in a large number of different volatiles have been observed when comparing urine mixtures of groups of an inbred wild-type strain and a congenic knock-out strain lacking functional MHC class I molecules. In contrast, more quantitative differences were observed between groups of the same inbred wild-type strain derived from different breeders [16] (for a review, see Kwak et al . [17] ). Hence, whereas variability in small airborne organic molecules may be important for recognition of individual scent owners [18] , [19] , physical evidence for an influence of the MHC on urinary volatiles remains elusive. The second mechanism calls attention to the immunological function of the MHC class I molecules as peptide-presenting proteins. MHC class I proteins are heterodimers composed of a polymorphic α chain and a conserved β chain (β 2 -microglobulin, β 2 m). Each classical MHC class I allele encodes a specific α chain that binds peptides according to its MHC motif which determines peptide length (usually 8–11 amino acids) and certain amino acids at two or three defined positions, called anchor residues [20] . MHC-bound peptides are otherwise variable. Co-expression of several alleles together with their respective sets of bound peptides provides an immunological signature for each individual. This immunological signature must be interpreted by the olfactory system. It is now well established that, in freely behaving mice, nonvolatile peptides gain access to sensory neurons of both the main olfactory system and the VNO during behavioural situations involving direct physical contact [21] , [22] , that such peptides are powerful ligands for subsets of vomeronasal and olfactory sensory neurons [21] , [22] , [23] , [24] , [25] (VSNs and OSNs, respectively), that they induce brain activity downstream from the sensory neurons in vivo [26] , and that synthetic MHC peptide ligands can be discriminated in social preference tests [22] and influence social learning and reproductive function in the context of the Bruce effect test [21] . However, it is important to note that there is also considerable evidence for the use of MHC-independent, individual identity signatures in mice in specific behavioural contexts [27] , [28] (but see the discussion in Ruff et al . [29] ). A major barrier preventing further progress in this field has been the lack of a source of natural MHC peptides accessible for nasal recognition. We hypothesized that mouse urine, which is sensed by the rodent nose in diverse behavioural contexts, contains peptides corresponding to ligands of self but not foreign MHC molecules. Therefore, we used genetically defined mouse strains to perform a partial characterization of the urinary peptidome employing mass spectrometry (MS). MS analysis shows the presence of abundant peptides with MHC motifs, but these peptides arise by MHC-independent mechanisms. Nonetheless, as demonstrated for a model peptide by a sensitive immunological assay, urine does contain MHC class I-dependent peptides in low concentrations, thus supporting the olfactory MHC peptide ligand hypothesis. Besides these differences, urinary peptide sequences show striking variations between mouse strains due to single-nucleotide and other genomic polymorphisms. Collectively, these results establish a molecular framework for the role of urinary peptides in conveying genome-related information to the olfactory system. We propose that such peptides could be used to transmit the degree of genetic disparity, for instance during interindividual interactions of sympatric species (cf. Chamero et al . [25] ), in addition to conveying MHC differences. Isolation and analysis of urinary peptides by mass spectrometry (MS) To search for genotype-specific differences in the urinary peptidome, we isolated peptides from the urine of different mouse strains and fractionated them by high-performance liquid chromatography (HPLC). A fraction expected to contain MHC ligands (as calibrated with the synthetic peptides SIIN F EK L and S Y FPEITH I ; anchor residues in bold) was subjected to MS ( Supplementary Fig. S1 and Supplementary Table S1 ). In an analysis with five mouse strains of the H2 b or H2 d haplotype (B10, B10.D2, B6, B6/β 2 m −/− and BALB/c, see Methods for details), we identified 639 peptides with a length between 7 and 32 amino acids. Selected groups of peptides with relevance for genotype-related individual differences will be categorized in the following paragraphs. Peptides with MHC binding motifs exist in mouse urine MHC peptide ligands occurring in urine in an MHC-dependent manner are expected to contain an MHC binding motif. 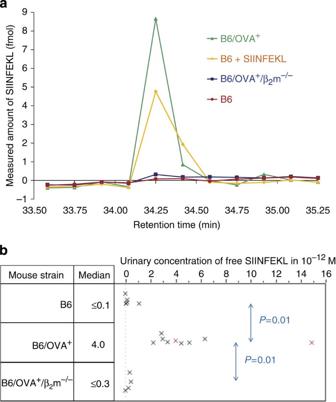Figure 1: HPLC fractions derived from urine are tested for the MHC model peptide SIINFEKL by ELISA. (a) A fraction of urine from a B6/OVA+mouse gives rise to a strong signal, while the corresponding preparations from a B6/OVA+/β2m−/−mouse and B6 mice are negative. Spiked synthetic SIINFEKL elutes at the same retention time as the substance detected in B6/OVA+urine. (b) SIINFEKL concentrations measured in the urine of individual B6/OVA+mice (n=9); there was no obvious correlation with the age of the mice (Supplementary Fig. S6). For comparison, results for individual B6/OVA+/β2m−/−(n=4) and B6 wild type (n=5) mice are shown. The two data points printed in red are derived from two separate urine samples of the same mouse. A two-tailed, heteroskedastic Student'st-test was applied with Bonferroni correction for two comparisons. To discover such peptides, we first scrutinized the ensemble of the 639 peptides for the presence of MHC binding motifs and discovered 17 peptides fitting to H2-K b , -D b , -K d or -L d motifs ( Table 1 and Supplementary Table S2 ). However, the urinary occurrence of these 17 peptides did not correlate with the MHC type of the mice, suggesting an MHC-independent production ( Supplementary Table S2 ). This conclusion was confirmed by a quantitative analysis of the five peptides that are marked in Table 1 . 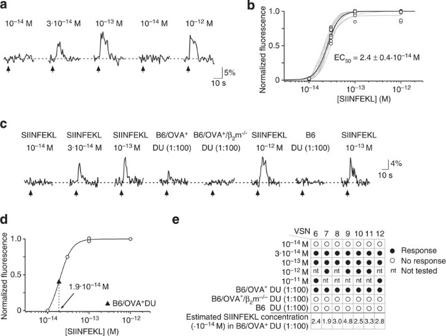Figure 2: Analysis of peptide and urine-evoked Ca2+responses in intact VSNs. (a) Example of somatic Ca2+recordings from a single VSN to different concentrations of SIINFEKL. A response is defined as a stimulus-dependent deviation in Ca2+fluorescence that exceeds twice the standard deviation of the mean of the baseline fluorescence noise. (b) SIINFEKL dose–response curves (grey) each recorded from a single VSN (n=12 cells, 8 slices). Relative changes in peak fluorescence (ΔF/F) induced by a given stimulus were normalized to the maximum peak response measured in a given VSN to construct a dose–response curve. The smooth curves (b,d) are fits of the Hill equation in combination with an iterative Levenberg–Marquardt nonlinear, least-squares fitting routine (chi-square test:P=0.96–0.99), defining threshold, EC50and saturation. The black curve represents the mean dose response curve; EC50value and SD are indicated. (c) Comparison of Ca2+responses in a single VSN to various concentrations of SIINFEKL and diluted urine (DU) obtained from B6/OVA+, B6/OVA+/β2m−/−and B6 mice. Repeated presentations indicate that Ca2+peak responses were highly reproducible and did not change over time under these conditions. (d) Estimating the active concentration of SIINFEKL in B6/OVA+urine (black triangle) from Ca2+responses of a single VSN to known concentrations of SIINFEKL. Same cell as inc. (e) Summary of response profiles of VSNs stimulated successively with SIINFEKL and different urine types as indicated. The SIINFEKL concentration in B6/OVA+DU estimated from the dose–response curve of each cell is indicated. Arrows indicate the time points at which stimulus application was turned on. Non-responders are not listed in the table. The examples listed in Table 2 show that the peptide LNSV F DQ L with an H2-K b motif (xxxx F / Y x(x)x L / M / I / V ) was present at a concentration of 3.5–10 × 10 −7 M, and the peptide TRVL N LGP I with an H2-D b motif (xxxx N xx(x)x M / I / L ) occurred at 1–4 × 10 −8 M. MHC motif peptides, like other urinary peptides, were derived from proteins of different locations in the body, most prominently from extracellular and membrane proteins typical for urine, blood and kidney ( Table 1 ). We also found extended forms of MHC motif peptides; for example, for TRVL N LGP I the longer versions IDQ TRVL N LGP I, TRVL N LGP I TR and SGNFIDQ TRVL N LGP I TR occurred, pointing to a gradual proteolytic generation. Table 1 Urinary peptides with MHC class I binding motif. Full size table Table 2 Urinary concentrations of two peptides with MHC class I binding motif and their extended versions. Full size table Two of these peptides, LNSVFDQL and TRVLNLGPI, were tested for their ability to bind to MHC class I molecules using an assay based on the peptide-induced stabilization and thereby increase of MHC molecules on the surface of RMA-S cells (H2 b haplotype) [30] , [31] . As expected, LNSV F DQ L showed binding to H2-K b and TRVL N LGP I did assemble with H2-D b molecules ( Supplementary Methods and Supplementary Fig. S2 ). Together, these results provide clear evidence for the existence of a pool of MHC motif peptides in urine that is independent of MHC expression and, therefore, these peptides cannot transmit information on the MHC type of an individual. For the reasons detailed below, the detection of bona fide MHC-dependent peptides by MS is not straightforward. Peptides in urine with single-amino-acid variations We asked if our set of peptides contains information about individuality apart from the MHC and considered the possibility that strain-specific differences in peptide sequences may occur as a result of genomic nucleotide variations. Accordingly, we searched the dbSNP database [32] for non-synonymous single-nucleotide variations affecting the sequence of urinary peptides by the exchange of single amino acids. Out of the 639 peptides, at least 47 (>7%) turned out to be encoded only in some but not all laboratory or wild-derived inbred mouse strains ( Supplementary Tables S4 and S7 ). Predicted peptides with single-amino-acid variations (SAVs) occur even within related inbred strains of mice, for example, within the C57 lineage, but are especially frequent between mice of different Mus musculus subspecies ( Supplementary Table S8 ). Importantly, at least four SAVs of urinary peptides were also anticipated to differ between B6 and BALB/c mice. 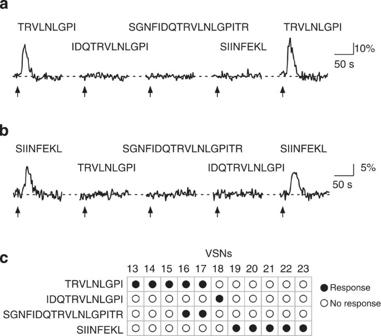Figure 3: Comparison of VSN Ca2+responses to stimulation with MHC-dependent and –independent peptides. (a,b) Examples of Ca2+responses from single VSNs to the MHC-independent MHC motif peptide TRVLNLGPI, its longer versions IDQTRVLNLGPI and SGNFIDQTRVLNLGPITR, and the MHC-dependent peptide SIINFEKL using saturating concentrations (10−11M). Arrows indicate the time points at which stimulus application was turned on. (c) Summary of response profiles from VSNs that were stimulated successively with TRVLNLGPI, IDQTRVLNLGPI, SGNFIDQTRVLNLGPITR and SIINFEKL. The results from repeated stimulations were identical. Note that there was no overlap between VSNs activated by TRVLNLGPI or SIINFEKL. By including these amino-acid sequence variations in the bioinformatical processing of our MS spectra, several B6-BALB/c-discriminating SAV peptide pairs could be identified ( Table 3 and Supplementary Methods ) and their distribution corresponded exactly to the nucleotide variations encoded in these mice, with B10 mice being more related to B6 than to BALB/c mice. For example, at position 398 of serine protease inhibitor A3K, a blood plasma protein, B6J and B10J mice encode an isoleucine whereas BALB/cJ mice encode phenylalanine. Accordingly, we detected the resulting urinary peptide I VIYHTSAQSIL only in mice of B6 or B10 background and the corresponding SAV form F VIYHTSAQSIL only in BALB/c mice ( Table 3 and Supplementary Tables S4, S5 and S8 ). The urinary concentration of SAV peptides is in the same order of magnitude (≤10 −6 M) as the MHC motif peptides described above. This is demonstrated by the fact that they are readily detected by MS and, more accurately, by the quantification of LNSV F D Q L ( Table 2 ), an MHC motif peptide of both B6 and BALB/c mice, which is encoded as LNSV F D R L in Mus musculus musculus ( Kap gene coding for kidney androgen-regulated protein, dbSNP accession number rs31887216; see Supplementary Tables S4 and S8 ). Table 3 Identified urinary peptides that are encoded in the genome of BALB/c but not B6 mice or vice versa. Full size table Further genomic variations influence urinary peptides Amino-acid variations in urinary peptides are expected to increase with growing taxonomic divergence. To demonstrate this, we aligned the 115 major urinary protein (MUP)-derived peptides that we identified in urine to the MUP sequence of Mus macedonicus , a species able to produce fertile F 1 females with the sympatric M. musculus [33] . In M. macedonicus urine contains only a single MUP, whereas the urine of M. musculus contains multiple different MUPs encoded by several paralogous genes [34] . Accordingly, out of the 115 MUP-derived peptides identified in urine, 58 are not encoded in the M. macedonicus MUP, including several peptides predicted to differ in more than three amino-acid residues between these two species ( Supplementary Fig. S3 ). Even within M. musculus , MUPs are a highly polymorphic group of proteins [35] and quantitative differences in urinary concentrations can occur in addition to qualitative ones. For example, the proportion of MUP20 (also known as darcin) among all MUPs is only <0.5% in male BALB/c but about 15% in male B6 mice [19] . Consequently, we found unique peptides from MUP20 more frequently and more abundantly in male urine of B6 than BALB/c origin ( Supplementary Tables S9 and S10 ). Females do not express MUP20 [19] , [36] and, thereby, unique MUP20-derived urinary peptides are both sex specific and vary in concentration in male urine. Genes with allele-specific occurrence or functionality can affect MUPs [36] as well as other proteins. Correspondingly, we identified 21 peptides derived from meprin A α (see Supplementary Table S11 ), a urinary metalloendopeptidase lacking mRNA expression in C3H/He mice (Fig. 5 in Jiang et al . [37] ). The urine of some other inbred strains also lacks meprin A α and the nonfunctional mep1a allele is genetically linked to the H2-k haplotype [38] , [39] . Mice deficient in this protein will not only lack the peptides encoded by mep1a but could also have a changed proteolytic cleavage pattern of urinary peptides. The effect of meprin A α deficiency should be considered when comparing mice of the H2-k haplotype with MHC congenic individuals in potentially MHC-related behaviours. Detection of an MHC-dependent peptide in mouse urine We were not able to detect MHC-dependent peptides, that is, those that are only present in the urine of mice expressing the corresponding MHC class I protein complex, by our MS approach (see above). Assuming that bona fide MHC-dependent peptides were present at very low concentrations, we reasoned that they would be missed in MS analyses due to the presence of a multitude of other, more abundant peptides. In fact, control experiments showed that a synthetic MHC peptide spiked into urine is not reproducibly detected at concentrations below 10 −11 M. Therefore, we developed a highly specific model system based on the well-studied H2-K b -presented peptide SIINFEKL corresponding to amino-acid residues 257–264 of chicken ovalbumin (OVA) [40] , [41] . The transgenic mouse line B6/OVA + expresses a cell surface protein composed of the entire chicken ovalbumin sequence and a transmembrane sequence under the control of the chicken β-actin promoter in all organs. Ovalbumin is naturally processed in this strain, resulting in SIINFEKL-H2-K b complexes [42] . B6/OVA + mice were crossed with B6/β 2 m −/− mice [43] , resulting in the strain B6/OVA + /β 2 m −/− , which produces ovalbumin but lacks the expression of functional MHC class I molecules (for a phenotypic characterization of lymphocytes isolated from these mouse strains see Supplementary Fig. S4 ). As a sensitive reagent for detecting SIINFEKL, we used the monoclonal antibody 25-D1.16, which is specific for the C-terminal residues of this peptide in association with H2-K b (ref. 44 ). We developed an enzyme-linked immunosorbent assay (ELISA) based on recombinant H2-K b -molecules refolded in vitro in the presence of the human β 2 m-subunit and the peptide TEYGFLNL. This assay can be used with [45] or without removing the bound peptide at alkaline pH before loading of SIINFEKL, the latter mode being about three times more sensitive ( Supplementary Fig. S5 ). Representative results of this assay performed on HPLC fractions of free urinary peptides (not bound to carrier molecules) from three mouse strains and a sample of B6 urine spiked with 5 × 10 −12 M SIINFEKL are shown in Fig 1a . B6/OVA + mice gave rise to a peak at the same retention time as the spiked peptide. Importantly, SIINFEKL was not detectable in B6/OVA + /β 2 m −/− and B6 mice. Therefore, the appearance of this peptide in urine requires the expression of both the protein of origin and the cognate MHC class I molecule as is the case for cellular MHC ligands [46] . Urine from B6/OVA + mice contained a median concentration of 4 × 10 −12 M SIINFEKL ( Fig. 1b ). This amount was present in free form because it was not retained by the 3-kDa ultrafilter used as a first step for peptide purification. The corresponding concentration detected in B6/OVA + /β 2 m −/− and B6 urine was ≤0.1 × 10 −12 M and ≤0.3 × 10 −12 M, respectively ( Fig. 1b ). By eluting peptides from potential carrier molecules using 20% acetonitrile [47] at pH 2, the fraction of SIINFEKL bound to undefined high-molecular-weight components was determined as 10–35% of the total urinary SIINFEKL. Figure 1: HPLC fractions derived from urine are tested for the MHC model peptide SIINFEKL by ELISA. ( a ) A fraction of urine from a B6/OVA + mouse gives rise to a strong signal, while the corresponding preparations from a B6/OVA + /β 2 m −/− mouse and B6 mice are negative. Spiked synthetic SIINFEKL elutes at the same retention time as the substance detected in B6/OVA + urine. ( b ) SIINFEKL concentrations measured in the urine of individual B6/OVA + mice ( n =9); there was no obvious correlation with the age of the mice ( Supplementary Fig. S6 ). For comparison, results for individual B6/OVA + /β 2 m −/− ( n =4) and B6 wild type ( n =5) mice are shown. The two data points printed in red are derived from two separate urine samples of the same mouse. A two-tailed, heteroskedastic Student's t -test was applied with Bonferroni correction for two comparisons. Full size image VSNs detect SIINFEKL and MHC-independent MHC motif peptides We next assessed whether naturally occurring peptides are detected by VSNs. We used acute VNO tissue slices of B6 mice and high-resolution confocal microscopy to image cellular Ca 2+ responses to peptide or urine stimulation [21] , [23] , [48] . Our previous findings have already established that synthetic MHC peptides are powerful ligands for V2R-expressing VSNs located in the Gαo-expressing layer of the VNO [21] , [23] , [24] , that a given peptide is detected by more than one V2R receptor [23] and that single amino-acid exchanges within peptides can be distinguished by VSNs [23] . Here, we asked whether individual VSNs are capable of detecting SIINFEKL at relevant concentrations. We recorded Ca 2+ responses in VSNs that recognized SIINFEKL and determined dose–response relationships in these cells ( n =12; Fig. 2a ). These curves revealed an EC 50 value of 2.3±0.4 × 10 −14 M ( n =12), demonstrating that these cells have an exquisite sensitivity for SIINFEKL. To determine whether SIINFEKL-selective VSNs are also activated by natural MHC peptides in urine, we stimulated these cells successively with diluted urine (1:100) obtained from B6/OVA + , B6 or B6/OVA + /β 2 m −/− mice. We searched specifically for VSNs responding to SIINFEKL but not to B6 urine to exclude unspecific responses of the neurons to compounds (including LNSVFDQL and TRVLNLGPI) present in urine of the B6 background strain. All VSNs selected in this manner responded to B6/OVA + but not to B6/OVA + /β 2 m −/− urine ( n =7; Fig. 2c–e ), demonstrating that the activity required expression of MHC class I and ruling out that the responses were caused by MHC-independent urinary peptides. Figure 2: Analysis of peptide and urine-evoked Ca 2+ responses in intact VSNs. ( a ) Example of somatic Ca 2+ recordings from a single VSN to different concentrations of SIINFEKL. A response is defined as a stimulus-dependent deviation in Ca 2+ fluorescence that exceeds twice the standard deviation of the mean of the baseline fluorescence noise. ( b ) SIINFEKL dose–response curves (grey) each recorded from a single VSN ( n =12 cells, 8 slices). Relative changes in peak fluorescence (Δ F / F ) induced by a given stimulus were normalized to the maximum peak response measured in a given VSN to construct a dose–response curve. The smooth curves ( b , d ) are fits of the Hill equation in combination with an iterative Levenberg–Marquardt nonlinear, least-squares fitting routine (chi-square test: P =0.96–0.99), defining threshold, EC 50 and saturation. The black curve represents the mean dose response curve; EC 50 value and SD are indicated. ( c ) Comparison of Ca 2+ responses in a single VSN to various concentrations of SIINFEKL and diluted urine (DU) obtained from B6/OVA + , B6/OVA + /β 2 m −/− and B6 mice. Repeated presentations indicate that Ca 2+ peak responses were highly reproducible and did not change over time under these conditions. ( d ) Estimating the active concentration of SIINFEKL in B6/OVA + urine (black triangle) from Ca 2+ responses of a single VSN to known concentrations of SIINFEKL. Same cell as in c . ( e ) Summary of response profiles of VSNs stimulated successively with SIINFEKL and different urine types as indicated. The SIINFEKL concentration in B6/OVA + DU estimated from the dose–response curve of each cell is indicated. Arrows indicate the time points at which stimulus application was turned on. Non-responders are not listed in the table. Full size image Using the VSN responses to known concentrations of SIINFEKL as a calibration, we estimated a SIINFEKL concentration of 2.9 × 10 −14 ±0.9 × 10 −14 M in 100-fold diluted urine ( n =7; Fig. 2d ). Taking into account the dilution factor, this value is in close proximity to the measured 4 × 10 −12 M in undiluted urine employing the ELISA ( Fig. 1b ). Together, these results show that subsets of VSNs are indeed capable of detecting an in vivo produced, bona fide MHC-dependent peptide at biologically relevant concentrations and within the urinary background of many other peptides. We also investigated VSN Ca 2+ responses to the MHC-independent MHC motif peptide TRVL N LGP I , together with two of its extended forms, IDQTRVLNLGPI and SGNFIDQTRVLNLGPITR, both of which are also detected in urine by MS. VSNs were successively stimulated with each of these peptides and with SIINFEKL (all at 10 −11 M). Cells that detected TRVLNLGPI were readily identified and an occasional response to some of the longer forms was also observed. However, there was no overlap between those cells that detected TRVLNLGPI or SIINFEKL ( Fig. 3 ), again illustrating the remarkable peptide specificity of VSNs. Figure 3: Comparison of VSN Ca 2+ responses to stimulation with MHC-dependent and –independent peptides. ( a , b ) Examples of Ca 2+ responses from single VSNs to the MHC-independent MHC motif peptide TRVLNLGPI, its longer versions IDQTRVLNLGPI and SGNFIDQTRVLNLGPITR, and the MHC-dependent peptide SIINFEKL using saturating concentrations (10 −11 M). Arrows indicate the time points at which stimulus application was turned on. ( c ) Summary of response profiles from VSNs that were stimulated successively with TRVLNLGPI, IDQTRVLNLGPI, SGNFIDQTRVLNLGPITR and SIINFEKL. The results from repeated stimulations were identical. Note that there was no overlap between VSNs activated by TRVLNLGPI or SIINFEKL. Full size image VSNs detect and discriminate SAV peptides Finally, we measured VSN Ca 2+ responses to the two SAV peptides I VIYHTSAQSIL and F VIYHTSAQSIL, which are not expected to bind to MHC class I molecules in their full 12-mer length and whose SAV position is unrelated to MHC anchor positions. As shown in Fig. 4 , the VNO indeed contains VSNs that are specific for either of these peptides or react with both (all at 10 −11 M). Hence, naturally occurring 12-mer SAV peptides are recognized by VSNs and an MHC motif is required neither for activation of these cells nor for their capability to discriminate between these ligands. 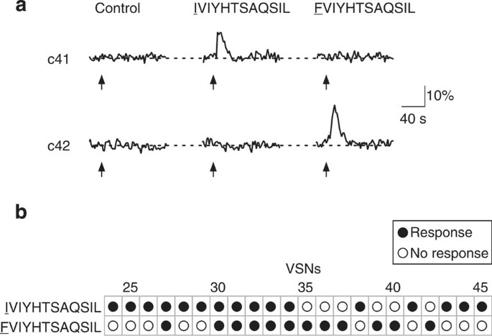Figure 4: VSNs detect and discriminate urinary SAV peptides differing in a single amino acid. (a) Example of Ca2+responses from single VSNs (c41 and c42) responding to either SAV peptide IVIYHTSAQSIL (10−11M) or FVIYHTSAQSIL (10−11M). Each peptide response was repeated at least once to demonstrate reproducibility (not shown). Increasing the concentration to 10−9M did not increase the number of responding cells and caused activation of the same VSNs that responded to 10−11M (not shown). Arrows indicate the time points at which stimulus application was turned on. (b) Summary of the response profiles from 22 VSNs stimulated successively and in random order with IVIYHTSAQSIL (10−11M) and FVIYHTSAQSIL (10−11M). Figure 4: VSNs detect and discriminate urinary SAV peptides differing in a single amino acid. ( a ) Example of Ca 2+ responses from single VSNs (c41 and c42) responding to either SAV peptide IVIYHTSAQSIL (10 −11 M) or FVIYHTSAQSIL (10 −11 M). Each peptide response was repeated at least once to demonstrate reproducibility (not shown). Increasing the concentration to 10 −9 M did not increase the number of responding cells and caused activation of the same VSNs that responded to 10 −11 M (not shown). Arrows indicate the time points at which stimulus application was turned on. ( b ) Summary of the response profiles from 22 VSNs stimulated successively and in random order with IVIYHTSAQSIL (10 −11 M) and FVIYHTSAQSIL (10 −11 M). Full size image This study provides a molecular basis for the evaluation of genotype by nasal chemosensory neurons. By analysing the identity and genomic origin of naturally occurring peptides in mouse urine, we have discovered multiple, partly overlapping peptide pools that contain distinct types of information related to genomic individuality. We have identified a novel family of MHC-independent peptides that differ in strains by single amino-acid exchanges, and we show for the first time (see Supplementary Note 1 ) that a bona fide MHC peptide ligand exists in urine in an MHC-dependent manner at biologically relevant concentrations. Hence, the emerging picture is a complex scenario in which multiple peptide families together with previously characterized MUPs [35] , [49] , [50] , formylated and maternally inherited peptides (not yet shown to exist in urine) [25] and possibly other yet undiscovered ligand families link the genotype of an individual with nasal chemoreception mechanisms. Future research should examine the contribution of these peptides to genotype discrimination in diverse behavioural contexts, but it will be essential to select urine samples for such experiments with care. For example, β 2 m −/− mice will not only lack MHC class I-dependent peptides but also peptides derived from the β 2 m protein, itself a prominent component of urine ( Supplementary Note 2 ). Our work fills a critical gap in the hypothesis that MHC peptide ligands may serve as signals of individuality in mice. We demonstrate that a prototypic MHC class I peptide ligand is present in urine in an MHC-dependent manner at a concentration of 4 × 10 −12 M largely in a free form that is considered to be responsible for neuronal stimulation (cf. Supplementary Note 3 ). We infer that other endogenously processed, but wild-type-encoded MHC-dependent peptides are likely present in urine in similar or even lower concentrations although they cannot be detected by today’s MS. The urinary concentrations of all MHC-dependent peptides may add up to approximately 10 −10 to 10 −8 M if one assumes that SIINFEKL represents between 0.1 and 10% of the H2-K b ligands [51] , [52] . In order for these peptides to qualify as pheromone-like cues that influence behaviour, a mouse must be able to recognize the qualitative difference of the MHC-dependent peptidome in the presence of the plethora of other, much more abundant urinary peptides. Subsets of VSNs are characterized by their extreme sensitivity for naturally occurring MHC peptide ligands (10 −14 –10 −12 M, cf. Leinders-Zufall et al . [21] , [23] and Fig. 2 ) and their remarkable specificity, which enables them to differentiate between urine from β 2 m-positive B6/OVA + and that from B6/OVA + /β 2 m −/− mice ( Fig. 2 ). We found VSNs that could specifically detect urinary SIIN F EK L in the presence of at least one abundant MHC motif peptide (LNSV F DQ L ) containing exactly the same anchor residues. Therefore, the recognition of MHC peptide ligands must also involve amino acids apart from the classical MHC anchor positions (cf. Leinders-Zufall et al . [23] ), that is, some VSNs do not seem to recognize all peptides bearing the same MHC anchor residues as a single entity. So far, evidence that MHC ligands serve as signals in the sensory evaluation of genotype rests on studies of the pregnancy block, which have shown that three synthetic peptides (each at 10 −4 M) of foreign but not self MHC type in the presence [21] , [53] or absence of urine [53] result in pregnancy failure. A key finding of our work is that MHC-independent peptides with MHC binding motif can be readily identified in urine and, as shown for representative examples, not only bind to the respective MHC molecules on cells but also stimulate VSNs with high specificity. These peptides occur at concentrations up to 6 orders of magnitude higher than SIINFEKL. Furthermore, N- and C-terminally extended versions of these peptides present in urine are also able to stimulate VSNs. Such peptides are generally not observed for peptides loaded onto MHC class I molecules via the antigen presentation pathway because extended forms are normally subject to rapid intracellular degradation [46] , [54] . Therefore, many urinary peptides with MHC motif are likely produced pre-renally, post-renally or both by proteases such as the metalloendopeptidases meprin A α and β that are found in the brush border of kidney proximal tubules and in secreted form in urine [39] . Notably, the detectable SIINFEKL is not produced by this mechanism because it was not found in the urine obtained from B6/OVA + /β 2 m −/− mice. Peptides with SAVs occur with or without MHC motif at urinary concentrations readily detectable by MS. As demonstrated with a 12-mer SAV peptide pair ( Fig. 4 ), an MHC motif is required neither for stimulation of specific VSNs nor for their capability to differentiate between SAVs. Therefore, most if not all urinary peptides of a suitable length (comprising at least the range between 3 (ref. 23 ) and 18 amino acids ( Fig. 3 )) may contribute to the individual peptide pattern detected by the ensemble of VSNs. Apart from peptides with differences in single amino acids, variations in urinary peptide composition can also arise from non-functional or multiplicated protein-coding genes, as exemplified for peptides derived from the metalloendopeptidase meprin A α or from MUPs. Therefore, SAV peptides and other MHC-independent urinary peptides contain sufficient information on genotype to enable discrimination of subspecies and sympatric species of M. musculus . Genotype discrimination via these peptides could be evolutionarily advantageous in a variety of processes ranging from assortative and disassortative mating to sympatric speciation. Importantly, SAV peptides will provide a signature of genomic individuality also in species lacking MUP polymorphism (for example, M. macedonicus ) and, because peptides can additionally be detected by the main olfactory epithelium [22] , they may even play a role in species lacking a VNO. Despite all the differences in urinary peptides, one should be aware that, when comparing two given strains of M. musculus , most urinary peptides are shared (for example, our MS analyses showed that at least 70% of peptides identified in B6 mice were also present in BALB/c mice). The picture on the variability of urinary peptides emerging from this study is very similar to that described for urinary volatiles [16] . In natural wild populations, urinary peptide patterns will differ qualitatively and quantitatively between individuals. However, within an inbred strain, we do not expect qualitative differences but possibly some variation in peptide abundance. Qualitative as well as quantitative differences will increase with decreasing evolutionary relatedness, that is, in the order: a given inbred strain (taken as reference)<sub-strains of this inbred strain<congenic strains (derived decades ago)<independently derived inbred strains≤subspecies of M. musculus <different species. Given that subsets of nasal chemosensory neurons exhibit a remarkable ability to differentiate a wide variety of peptides, the urinary peptide pattern represents a real-time sampling of the expressed genome available for chemosensory assessment by other individuals. Animals used as urine donors C57BL/6J mice (abbreviated B6, stock #000664) and mice with a targeted mutation in the β 2 -microglobulin gene (B6.129P2- B2m tm1Unc J, abbreviated B6/β 2 m −/− , stock #002087) were obtained from the Jackson Laboratories, Bar Harbor, Maine. Mice homozygous for the B2m tm1Unc mutation have little, if any, MHC class I protein expression on the cell surface, and there are few CD8 + cytotoxic T-cells. The mutation was originally produced by Koller et al . [43] in strain 129. Backcrossing for 11 generations to C57BL/6J mice at the Jackson Laboratories ensures that nearly all loci are of C57BL/6J origin. Strain C57BL/6-Tg(ACTB-OVA)916Jen/J (abbreviated B6/OVA + , stock #005145) is a transgenic line produced in B6 mice, which expresses chicken ovalbumin as a transmembrane protein on cell surfaces of all organs [42] . This strain was expanded by crossing breeders obtained from the Jackson Laboratories. Strain B6/OVA + /β 2 m −/− was produced by mating B6/β 2 m −/− and B6/OVA + mice; all F1 animals expressed ovalbumin. Derived F2 animals were typed for ovalbumin and the presence of CD8 + T lymphocytes. OVA + mice lacking CD8 + T-cells were designated B6/OVA + /β 2 m −/− (see Supplementary Fig. S4 for details). For MS experiments, mice of strains C57BL/10SnJ (abbreviated B10, stock #000666), B10.D2- Hc 1 H2 d H2-T18 c /nSnJ (abbreviated B10.D2, stock #000463) and BALB/cJ (stock #000651) were used in addition to B6 and B6/β 2 m −/− animals. All B6-derived mice as well as B10 mice carry the H2 b haplotype. BALB/c mice express the H2 d haplotype; the congenic line B10.D2 carries the H2 d complex on the background of B10. For each of the five strains used in MS analyses, we pooled urine from four to five individuals in order to diminish the influences of intra-strain variability. All mice were males aged 3–25 months (for details, see Supplementary Fig. S6 and Supplementary Table S1 ). They were kept singly and obtained food and water ad libitum . Mice for MS analyses were fed with a defined composition diet (C1000 Control Diet Rats/Mice, Altromin, Lage, Germany) containing bovine milk protein as the only protein source to control for urinary peptide contaminants from food. Isolation of urinary peptides Urine was collected individually either by holding the animals over small plastic petri dishes and freezing urine immediately in dry ice (for the data in Figs 1 and 2 , Table 2 and Supplementary Fig. S6 ) or with the help of metabolic cages (for the data in Tables 1 and 3 , Supplementary Figs S1, S3 and S7–S46 and Supplementary Tables S2–S11 ). Isolation and fractionation of urinary peptides for analysis by MS and ELISA is described in Supplementary Methods . Mass spectrometry The HPLC fraction of interest, comprising 4 min (one experiment with 10 s fraction), was concentrated using lyophilization and/or vacuum centrifugation. We then purified the concentrate on a C 18 StageTip [55] . Peptides were eluted with 80% acetonitrile/0.5% acetic acid. The eluate was concentrated in a vacuum centrifuge, supplemented with 1/10 volume 2% acetonitrile/1% TFA and loaded on a 15 cm × 75 μm nano-HPLC column packed in-house with 3 μm C 18 beads (Dr. Maisch GmbH). Peptides were eluted using a gradient of 16–40% acetonitrile in 0.5% acetic acid within 97 or 105 min. We applied a nanoLC-2D (Eksigent) or an Easy-LC (Proxeon Biosystems) nano-HPLC system coupled to an LTQ Orbitrap XL mass spectrometer (Thermo Fisher Scientific). Parent ions were recorded in the Fourier transform (FT)-Orbitrap mass analyser at a resolution of 60,000; fragment ions were either generated by collision-induced dissociation and measured in the linear trap quadrupole (LTQ) or produced by higher-energy collisional dissociation and recorded in the FT-Orbitrap mass analyser. MS data were analysed with the MaxQuant software [56] version 1.0.14.3 utilizing Mascot (Matrix Science) as a search engine for peptide identifications. The search strategy employed a target-decoy protein database including the international protein index (IPI) for M. musculus , commonly observed contaminants and reversed sequences. The false discovery rate was set to ≤1% in MaxQuant. Additionally, we confined the results to those peptides that had been identified at least once with a Mascot score ≥25. Employing dbSNP [32] XML files (revision 14 April 2010) we bioinformatically screened the 639 identified peptides for those predicted to contain SAVs. More details about MS analyses, SAV peptide identification and peptide sequence verification are given in Supplementary Tables S1, S3, S5, S6, S10, S11 , Supplementary Figs S7–S46 and Supplementary Note 4 . ELISA for the determination of SIINFEKL The common 400 μl well enzyme-linked immunosorbent assay (ELISA) format was not sensitive enough to detect SIINFEKL in HPLC fractions derived from 5 ml urine of individual B6/OVA + mice. Therefore we employed a miniaturized ELISA based on capillary forces (IMAPlate 5RC96, NCL New Concept Lab, Moehlin, Switzerland [57] ). This enabled us to take up lyophilized HPLC fractions in a final volume as small as 17 μl RPMI 1640/1% BSA containing (NH 4 ) 2 CO 3 to reach pH≈7.5 for triplicate measurements. All incubations, except blocking, were done in a moist chamber by contact-free insertion of the IMAPlate into an empty, flat-bottomed, 400-μl-well ELISA plate. For all washings we applied 50 μl/well phosphate-buffered saline/1% bovine serum albumin/0.05% Tween 20 (PBS/BSA/Tween) from the top of the plate. Coating was performed by dipping the IMAPlate into 36 ml 0.05 M Na 2 CO 3 /NaHCO 3 , pH 9.6, containing 5 μg/ml streptavidin in a reagent dish (cover of an ELISA plate; incubation for 30 min at 37 °C). After two washings, the IMAPlate was blocked by putting it into a reagent dish with 70 ml PBS/BSA/Tween for 1 h at room temperature (RT). From the top of the plate we then loaded 15 μl/well biotinylated H2-K b complex (6 μg/ml in PBS/BSA/Tween, produced in house using the H2-K b peptide TEYGFLNL for refolding [58] ) and incubated at 7 °C overnight. The plate was washed twice and 5 μl of SIINFEKL standards in RPMI 1640/1% BSA or HPLC fractions were pipette-loaded into individual wells from the bottom side of the plate and incubated at RT for approximately 2 h. After two washings the SIINFEKL-H2-K b -complex was detected using the monoclonal antibody 25-D1.16 (in-house-produced hybridoma supernatant, 1/5 in PBS/BSA/Tween). We either pipette-loaded 5 μl/well from the bottom side or 15 μl from the top side of the plate, incubated for 1 h at RT and washed twice. Horseradish peroxidase-coupled goat anti-mouse IgG1 antibody (SouthernBiotech) was dissolved 1/5000 in 12 ml PBS/BSA/Tween in a reagent dish and loaded by dipping. Incubation on ice for 30–60 min and three washings followed. Twelve millilitres each of TMB Peroxidase Substrate and Peroxidase Substrate Solution B (KPL, Gaithersburg, USA) were mixed in a reagent dish and applied to the IMAPlate by dipping. The colour reaction was stopped by dipping the plate briefly in 85% H 3 PO 4 and subsequent inversion until the acid had distributed in the wells. Absorbance was measured at 450 nm with a SpectraMax 340 ELISA reader (Molecular Devices, Munich) and corrected for absorbance at 650 nm. VSN Ca 2+ imaging Imaging experiments were performed in coronal VNO tissue slices freshly prepared from C57BL/6 mice (2–6 months old, either sex). In wild-type mice, ~1% of all VSNs respond to a given peptide [21] , [23] . We imaged and analysed >6,000 VSNs in 31 slices from 20 mice using the methods described previously [21] , [23] , [48] . Briefly, mice were euthanized using CO 2 followed by decapitation. The two VNOs were quickly removed and submerged in oxygenated extracellular solution 1 (95% O 2 / 5% CO 2 ) containing (in mM): 120 NaCl, 25 NaHCO 3 , 5 KCl, 5 BES, 1 MgSO 4 , 1 CaCl 2 , 10 glucose (300 mOsm). The vomer bones were then removed, the VNO was embedded in 3% low-gelling temperature agarose and coronal slices (250 μm) were cut on a vibratome (Microm HM 650V). Slices were loaded with the Ca 2+ indicator fluo-4/AM (Invitrogen) and imaged using a laser scanning confocal system. Optical sections were approximately 10 μm thick. All scanning head settings except gain (that is, black level, detector aperture and laser neutral density filter) were kept constant during each experiment. The gain was usually adjusted slightly, but only once at the beginning of an experiment during acquisition of baseline images. Images were acquired at 0.5 Hz using LaserSharp2000 software (Zeiss) and analysed using NIH ImageJ and Igor Pro software (Wavemetrics). Regions of interest corresponding to the somata of single VSNs were outlined and the average pixel values in these regions were measured. These somatic fluorescence changes (in arbitrary fluorescence units) are presented as absolute values (Δ F / F ) of the relative changes in fluorescence intensity (Δ F ) normalized to the baseline fluorescence ( F ), which was obtained prior to stimulation. As a sensitive criterion for a responding neuron, the stimulus-evoked fluorescence intensity had to exceed twice the standard deviation of the mean of the baseline fluorescence noise in a given time window after stimulus onset. All peptides and urine were diluted in HEPES-buffered extracellular solution 2 consisting of (in mM): 145 NaCl, 5 KCl, 10 Hepes, 1 MgCl 2 , 1 CaCl 2 , adjusted to pH 7.2 (NaOH) and 300 mOsm (glucose). Serial dilutions were made from the same stock solution. Each stimulus was added for 10 s to the superfusing bath solution (laminar flow chamber). All stimuli were delivered in random order. Interstimulus interval was fixed at 4 min to allow for recovery from adaptation [59] . How to cite this article: Sturm, T. et al . Mouse urinary peptides provide a molecular basis for genotype discrimination by nasal sensory neurons Nat. Commun. 4:1616 doi: 10.1038/ncomms2610 (2013).